Termination of the unfolded protein response is guided by ER stress-inducedHAC1mRNA nuclear retention Cellular homeostasis is maintained by surveillance mechanisms that intervene at virtually every step of gene expression. In the nucleus, the yeast chromatin remodeler Isw1 holds back maturing mRNA ribonucleoparticles to prevent their untimely export, but whether this activity operates beyond quality control of mRNA biogenesis to regulate gene expression is unknown. Here, we identify the mRNA encoding the central effector of the unfolded protein response (UPR) HAC1 , as an Isw1 RNA target. The direct binding of Isw1 to the 3’ untranslated region of HAC1 mRNA restricts its nuclear export and is required for accurate UPR abatement. Accordingly, ISW1 inactivation sensitizes cells to endoplasmic reticulum (ER) stress while its overexpression reduces UPR induction. Our results reveal an unsuspected mechanism, in which binding of ER-stress induced Isw1 to HAC1 mRNA limits its nuclear export, providing a feedback loop that fine-tunes UPR attenuation to guarantee homeostatic adaptation to ER stress. The maintenance of cellular homeostasis is ensured by stress-signaling pathways that constantly adapt gene expression programs to intra or extracellular perturbations. While failure to activate these pathways prevents stress adaptation, prolonged signaling can also culminate in cell death. Accordingly, the accumulation of unfolded proteins in the lumen of the ER, referred to as ER stress, initiates the conserved UPR that alleviates the stress [1] , and sustained or unresolved ER stress is detrimental to cell viability, both in mammalian [2] and yeast cells [3] , [4] . In yeast the UPR is signaled by a unique ER-localized receptor-like kinase and ribonuclease, Ire1 [5] , [6] (IRE1αβ in mammals). Activated Ire1 eliminates a 252-nucleotide translation inhibitory intron within the constitutively expressed and nuclear-exported mRNA encoding Hac1, a bZIP transcription factor [7] , [8] . This “RNA editing” event is completed by the tRNA ligase Rlg1 (RTCB complex in mammals) which ligates HAC1 exons [9] , thereby allowing its translation [7] , [10] . Hac1 is in turn imported into the nucleus, where it up-regulates expression of UPR target genes containing a conserved UPR element (UPRE) in their promoters, to relieve ER stress [11] . Because only the edited form of Hac1 is translated, this non-canonical cytoplasmic splicing event provides the key trigger of the signaling. On the other hand, the mechanisms that regulate UPR termination are less well established. Previous studies have nonetheless provided important insights into how Ire1 activity can be attenuated, by its binding to the UPR-induced ER-resident chaperone Kar2 (BiP in mammals) which buffers its oligomerization [12] , by its dephosphorylation [3] , [13] or by phosphoryl transfer within the Ire1 kinase [4] . However, little is known about the regulations that target HAC1 mRNA biogenesis beyond the control of its non-canonical splicing. Quality control (QC) of gene expression is known to be initiated in the nucleus, where multiple mechanisms scrutinize early steps of gene expression [14] , [15] , [16] . Specifically, nuclear mRNA biogenesis and export is precisely regulated so that only accurately packaged and processed mRNA ribonucleoparticles (mRNP) are exported to the cytoplasm. This is in part achieved through nuclear retention of immature mRNPs, which we recently reported to be initiated at the chromatin level by the nucleosome spacing-enzyme Isw1. This ATP-dependent chromatin remodeler contributes to the regular spacing and phasing of the nucleosomes over coding regions [17] . Although inactivation of ISW1 leads to global perturbation of chromatin organization -associated with increased intragenic cryptic transcription [18] and characterized by reduced nucleosome spacing [19] , [20] , [21] -it has little influence on cell growth and gene expression, typified by a modest derepression of very few genes [22] , [23] , [24] , [25] . Strikingly however, it promotes the release from chromatin and consecutive export of nuclear-retained mRNPs [26] . While this pathway was characterized using mRNP biogenesis mutants or reporter RNAs [26] , we speculated that it may operate in physiological conditions to proofread mRNA biogenesis and to regulate nuclear export of mRNA and thereby gene expression. Here we demonstrate that Isw1 nuclear RNA retention activity is crucial to fine-tune the UPR homeostatic feedback loop. By directly binding the 3′UTR of the HAC1 transcript, Isw1 limits its nuclear export and therefore cytoplasmic splicing. Under ER stress, UPR transcriptional induction of ISW1 fosters this nuclear mRNA retention activity, which is ultimately decisive for the accurate attenuation of this signaling pathway and for cell survival upon ER stress. Isw1 interacts with the 3′UTR of HAC1 We previously reported that Isw1 was able to directly interact with RNA, using in vivo UV cross-link followed by stringent purification of “zero-length” Isw1-RNA interactants [26] . We have now performed CRAC ( c rosslinking a nalysis of c DNA) experiments [27] , [28] to analyze the binding of Isw1 to its RNA targets (Fig. 1a , unpublished data). While the full genome-wide analysis of these experiments is beyond the scope of this report, we have identified that Isw1 binds the HAC1 mRNA (Supplementary Fig. 1a ), among others (Supplementary Fig. 1b ), and analyzed the corresponding reads. Inspection of these data suggested that Isw1 strongly binds to the 3′UTR of the transcript (Supplementary Fig. 1a ). This was confirmed by an Isw1 RNA immunoprecipitation (RIP) assay [26] including as a control, a strain expressing a chimeric version of HAC1 , in which its 3′UTR was replaced with that of ACT1 ( HAC1-3’ACT1 ) (Fig. 1b ). Whereas the same amount of a previously reported bona fide Isw1 RNA target (i.e. IOC2 ) was co-immunoprecipitated with Isw1 in cells expressing the wild-type (WT) or the chimeric version of HAC1 , the interaction of Isw1 with the HAC1 transcript was significantly decreased in HAC1-3’ACT1 cells compared to WT (Fig. 1b ), supporting the prominent role of the 3′UTR region of HAC1 in its interaction with Isw1. Fig. 1: Isw1 interacts with the 3’UTR of HAC1 mRNA. a Scheme depicting the identification of Isw1-bound transcripts by in vivo UV-crosslinking and analysis of cDNA. Growing yeast cells expressing dual affinity tagged (HIS6-TEV-PrA) Isw1 were UV-irradiated with 254 nm UV light to covalently crosslink RNA-protein complexes, which were immunopurified under stringent wash condition to prevent the recovery of indirect RNA targets. After ligation of linkers, crosslinked RNAs were converted to cDNA, PCR amplified, and sequenced. b The interaction between HAC1 mRNA and Isw1 is mediated by its 3′UTR. RIP assays were performed with HTP tagged Isw1 in cells expressing wild type HAC1 ( HAC1 3′UTR HAC1 ) or a chimeric HAC1 ( HAC1 3′UTR ACT1 ). Untagged WT cells were used as a negative control. The ratio of co-immunoprecipitated HAC1 or IOC2 RNA to total RNA relative to WT was quantified by qRT-PCR. n = 3 independent experiments, mean ± s.d. Unpaired one-tail t -test ( p values relative to No Tag: HAC1 , Isw1-HTP: 4.56E−04 HAC 1 -3′ ACT1 , Isw1-HTP: 9.95E−02 for HAC1 and Isw1-HTP: 2.89693E−06, HAC 1 -3′ ACT , Isw1-HTP: 3.55186E−05 for IOC2 ). Full size image ISW1 inactivated cells fail to terminate the UPR The association between Isw1 and the HAC1 mRNA prompted us to evaluate the contribution of this mRNA nuclear retention factor to the UPR. To this aim, we profiled the transcriptional UPR output in WT and ISW1 inactivated cells, during a time-course in which ER stress was induced by a two-hour treatment with tunicamycin (Tm), a well-characterized inhibitor of N-linked glycosylation that induces the accumulation of unfolded proteins in the ER. Tm treatment was followed by a wash of the drug from the medium, thereby allowing analysis of the activation and termination phases of the UPR [3] by qRT-PCR (Fig. 2a ). Monitoring HAC1 mRNA splicing using primers specific to the spliced ( i nduced, HAC1i ), unspliced ( HAC1u ) and total ( HAC1Tot ) forms of HAC1 revealed that Tm equally induced HAC1i formation in WT and isw1 Δ cells (Fig. 2b , compare untreated and Tm 2H). As previously reported, the level of HAC1 i declined gradually over time to reach its initial level four hours after Tm removal in WT cells, corresponding to an adaptive phase characterized by an adjustment of the ER capacity that correlates with Ire1 turn-off [3] , [4] , [12] . In contrast, the decrease of HAC1i was delayed in isw1 Δ cells and did not reset by four hours after Tm wash (Fig. 2b ). Consistently, the percentage of spliced HAC1 (Fig. 2c ) and the expression of Hac1 protein (Fig. 2d ) and Hac1 transcriptional targets (Fig. 2e , Supplementary Fig. 2a ) were significantly sustained after Tm removal in isw1 Δ compared to WT cells. Genome-wide expression profiling of these strains across similar UPR time-courses (Untreated- Tm 2 H- Wash 3 H) reinforced these conclusions. While in WT cells the expression fold change of UPR target genes relative to untreated conditions was significantly decreased three hours after Tm wash compared to two hours Tm treatment, it remained unchanged in isw1 Δ cells (Fig. 2f ). Accordingly, whereas 16 out of 25 of the most robustly induced UPR genes remained differentially expressed 3 h after Tm removal in isw1 Δ cells, only 3 of them maintained an induced state in WT cells (Supplementary Fig. 2b ). Importantly, Tm similarly induced the expression of UPR target genes [11] in WT and isw1 Δ cells (Supplementary Fig. 2c ) and only the attenuation of their expression upon Tm removal was reduced in isw1 Δ cells compared to WT. As such, differential UPR gene expression between WT and isw1 Δ cells was only observed 3 h after Tm removal (Supplementary Fig. 2d ). In addition, to exclude the possibility that the sustained UPR activation observed in isw1 Δ results from an impaired and therefore delayed UPR activation, we conducted a careful comparison of UPR induction after a 2 h Tm treatment in WT and isw1 Δ cells. The analysis of RNA Polymerase II (RNAPII) recruitment on 25 of the most robustly induced UPR target genes by ChIP-qPCR (Supplementary Fig. 2e ), as well as the genome-wide profiling of UPR transcription using the CRAC technique to detect the position of RNAPII on UPR targets, revealed that WT and isw1 Δ cells display comparable UPR induction profiles (Supplementary Fig. 2f, g ). Finally, these results were recapitulated when UPR was triggered using DTT, a reducing agent that causes protein misfolding in the ER by counteracting disulfide bonds formation (Supplementary Fig. 2h–k ). Thus, Isw1 is dispensable for HAC1 activation but necessary for accurate UPR abatement. Fig. 2: ISW1 inactivation prevents accurate UPR termination. a Tm UPR time course experimental setting: WT and isw1 Δ exponentially growing cells were treated with 1 μg/mL tunicamycin for 2 h, washed and resuspended in Tm free medium. Samples were collected at t = −2 h (Untreated), t = 0 (Tm 2 H), t = 1 h (Wash 1 H), t = 2 h (Wash 2 H), t = 3 h (Wash 3 H), and t = 4 h (Wash 4 H) for analysis of HAC1 mRNA splicing and expression of UPR target genes by qRT-PCR using the depicted primers. b qRT-PCR analysis of the expression levels of HAC1 i, HAC1 u, and HAC1 Tot relative to SCR1 or to WT, in WT and isw1 Δ cells during the Tm UPR time course depicted in b . n = 5 independent experiments, mean ± s.d. c HAC1 splicing is sustained in isw1 Δ compared to WT cells during Tm UPR time course. The percentage of spliced HAC1 ( HAC1 i / HAC1 Tot x100) was calculated from the values obtained in b . n = 5 independent experiments, mean ±  s.d. Unpaired one-tail t -test ( p values relative to WT: 4.20E−03 4.40E−01, 8.67E−02, 1.04E-03, 2.45E−03, 1.14E−02 for Untreated, Tm 2 H, Wash 1 H, Wash 2 H, Wash 3 H, Wash 4 H respectively). d Hac1 expression is sustained in isw1 Δ compared to WT cells. Total protein extracts from WT and isw1 Δ cells treated or not with 1 μg/mL Tm for 2 H were analyzed by western blot with anti-Hac1 and Pab1 (loading) antibodies. The level of Hac1 and Pab1 was quantified. n = 4 independent experiments, mean ± s.d. Unpaired one-tailed t -test ( p values relative to WT: 0.004387283, 0.039668848, 0.024072787 at Tm 2 H, Wash 2 H, Wash 3 H respectively). e The mRNA expression level of canonical Hac1 targets is prolonged in isw1 Δ cells compared to WT, as evaluated by qRT-PCR analysis of PDI1 transcript expression relative to SCR1 during Tm UPR time courses. n = 5 independent experiments, mean ± s.d. f Whisker plots of expression fold change (Log2 FC) for all UPR (defined in ref. 11 ) and non-UPR target genes at Tm 2 H and Wash 3 H relative to untreated in WT and isw1 Δ cells. Boxes extend from the 25th to 75th percentiles. The line in the middle of the box is plotted at the median. Whiskers are plotted down to the minimum and up to the maximum value, and each individual value is plotted as a point superimposed on the graph. n = 3 independent biological replicates. Paired two-tailed t -test ( p values for WT UPR targets <0.00001, for isw1 Δ UPR targets 0.1408, for WT non-UPR targets 0.053, for isw1 Δ non-UPR targets 0.1048). Full size image Cells lacking ISW1 are sensitive to ER stress and defective for ER homeostasis reset Examination of the physiological consequences of defective UPR attenuation uncovered that ISW1 inactivation sensitized cells to ER stress (Fig. 3a, b ), a phenotype reminiscent of ire1 mutants that activate the UPR in response to ER stress but are unable to turn-down their ribonuclease activity [3] , [4] . This unlikely resulted from an inability to translate UPR-induced mRNAs as no differences were observed, between WT and isw1 Δ cells, in the steady-state level upon Tm induction of Kar2, an ER Hsp70 and canonical UPR target (Supplementary Fig. 3a ). Combination of ISW1 inactivation to an ire1D828A mutation that impedes UPR abatement by mimicking an active RNase conformation [3] led to increased Tm sensitivity of the double mutant compared to each single mutant (Fig. 3b, c ), implying that Isw1 and Ire1 intervene in two independent pathways of UPR termination. This stress sensitivity phenotype was not general, as no difference in sensitivity to oxidative, osmotic or mitochondrial stress was observed between WT and isw1 Δ cells (Fig. 3d , Supplementary Fig. 3b ). To gauge how sustained UPR activation influences the ER folding capacity, we monitored, during Tm-time-courses, the glycosylation status of Protein disulfide isomerase (Pdi1), an ER-resident protein that supports protein folding by catalyzing disulfides. Pdi1 features N-glycosylation at five sites [29] , which can be abolished upon deglycosylation with PNGase, resulting in increased mobility of the protein by SDS PAGE (Supplementary Fig. 3c ). When glycosylation was inhibited for two hours with tunicamycin, Pdi1 was detected as two bands, corresponding to the glycosylated and unglycosylated forms of the protein, in both WT and ire1 Δ cells. In WT cells, upon removal of the drug and during the abatement phase of the UPR, Pdi1 progressively recovered its initial glycosylation status. In ire1 Δ cells, Pdi1 remained deglycosylated, reflecting the inability of cells that are unable to initiate the UPR to alleviate the stress (Supplementary Fig. 3d ). Strikingly, upon identical experimental settings, the kinetics of Pdi1 glycosylation was delayed in isw1 Δ and ire1D828A cells compared to WT (Fig. 3e ), an effect that was strengthened in isw1 Δ ire1D828A double mutant (Fig. 3f ). This delay is indicative of an altered restoration of the ER oxidative protein folding capacity. Thus, isw1 Δ and ire1D828A cells present improper UPR termination and increased sensitivity to ER stress accompanied with defective reestablishment of ER homeostasis. Fig. 3: ISW1 inactivated cells are sensitive to ER stress and defective for ER homeostasis reset. a isw1 Δ cells are more sensitive than WT to tunicamycin: fivefold serial dilutions of the indicated strains grown for 3 days at 30 °C on selective media containing (+ER stress) or not (−ER stress) 0.4 μg/mL or 0.6 μg/mL Tm. b Viability assay. Exponentially growing cells were treated or not with 1 μg/mL Tm for 24 H and stained with propidium iodide (PI). The percentage of PI negative cells is plotted. A minimum of 300 cells per condition were counted. n = 3 independent experiments, mean ± s.d. Unpaired one-tail t -test ( p values relative to WT Untreated: 0.445937983, 0.093299173, 0.110093567, 0.41523827 for isw1 Δ, ire1D828A, isw1 Δ ire1D828A and ire1 Δ respectively. p values relative to WT Tm: 0.000201098, 0.000243914, 2.46522E-05, 7.60488E-06 for isw1 Δ, ire1D828A, isw1 Δ ire1D828A and ire1 Δ respectively. p value for ire1D828A isw1 Δ relative to isw1 Δ 0.00662224. p value for ire1D828A isw1 Δ relative to ire1D828A 5.76554E-05. c isw1 Δ and ire1D828A mutations have compounding effects. Fivefold serial dilutions of the indicated strains grown for 3 days at 30 °C on selective media containing (+ER stress) or not (−ER stress) 0.4 μg/mL or 0.6 μg/mL Tm. d isw1 Δ cells are not more sensitive than WT cells to oxidative, osmotic and mitochondrial stresses. Fivefold serial dilutions of the indicated strains grown for 2 days at 30 °C with or without 2.5 mM H 2 O 2 , 0.5 M NaCl or 10 μM Carbonyl cyanide- p -trifluoromethoxyphenylhydrazone (FCCP), a potent uncoupler of mitochondrial oxidative phosphorylation. sod2 Δ, hog1 Δ and get1 Δ mutants respectively serve as positive controls for the effect of the stresses. e , f Pdi1 re-glycosylation during Tm UPR time course. Total protein extracts from WT, isw1 Δ, ire1D828A, and isw1 Δ ire1D828A cells collected during Tm UPR time courses were analyzed by western blot with anti-Pdi1 antibodies. Three independent experiments were performed with similar results. Full size image Expression of HAC1 splicing machinery, stability of HAC1 mRNA and kinetics of Ire1 cluster assembly and disassembly are unaffected by ISW1 inactivation We next investigated the molecular mechanism underlying the persistence of HAC1 splicing during the termination phase of the UPR. Transcriptional analysis indicated that the expression level of HAC1 mRNA splicing machinery ( IRE1 , RLG1 ) was unaffected by ISW1 inactivation (Supplementary Fig. 4a ). We then asked whether sustained HAC1 splicing could result from a stabilization of the HAC1 transcript consequent to ISW1 inactivation. Monitoring the stability of both forms of HAC1 mRNA following transcriptional inhibition in cells previously treated ( HAC1 i) or not ( HAC 1u) with DTT to allow for HAC1 i production (Supplementary Fig. 4b ) revealed that ER stress stabilized HAC1 u, in agreement with a previous report [30] (Supplementary Fig. 4c ). However, ISW1 inactivation did not affect the stability of either forms of HAC1 . Finally, we considered that the impaired UPR attenuation observed in isw1 Δ cells could be due to sustained Ire1 activation. To evaluate the kinetics of Ire1 activation and deactivation, we examined the kinetics of Ire1 clusterization and declusterization into foci, to which HAC1 mRNA is recruited upon UPR induction for optimal splicing and which disappear upon UPR abatement [31] , [32] , [33] , [34] , [35] , [36] . ISW1 inactivation did not alter the kinetics of Ire1 foci formation or dissociation (Supplementary Fig. 4d ) examined in strains expressing at similar levels (Supplementary Fig. 4e ) a GFP-tagged version of Ire1 that preserves its functions [31] . We concluded that the UPR termination defect detected in isw1 Δ cells does neither result from an increased expression of the “UPR splicing machinery” nor from a stabilization of the HAC1 transcript nor defective Ire1 deactivation. Isw1 is required for HAC1 mRNA nuclear retention Since Isw1 binds and retains transcripts in the nucleus [26] , we reasoned that its inactivation may influence the kinetics of HAC1 mRNA nuclear export. We therefore implemented “transcriptional chase” experiments in which the expression of HAC1 was turned off by the addition of the transcriptional inhibitor phenanthroline to the growth media. This allows to follow the fate of transcripts synthesized before transcription inhibition (t0, Fig. 4a ), by RNA Fluorescence In Situ Hybridization (FISH) using HAC1 exons-specific probes (Supplementary Fig. 5a ). As previously reported, the distribution of the HAC1 transcript was mainly cytoplasmic [37] , with a nuclear dot corresponding to its transcription site detected upon normal conditions. In WT cells, the percentage of cells displaying an accumulation of transcripts in this nuclear dot decreased during the course of the transcriptional inhibition, reflecting the export of the corresponding transcripts. Strikingly, this decrease was faster in isw1 Δ than in WT cells (Fig. 4b ), indicating that ISW1 inactivation fosters the release of nuclear retained HAC1 transcript from chromatin. To further strengthen this observation, we quantified, the intensities of the HAC1 mRNA signal in the nucleus and the cytoplasm of untreated cells, an approach that we validated on a manually quantified and previously published data set [26] (Supplementary Fig. 5b ) as well as by evaluating the number of cytoplasmic HAC1 transcripts through manual counting (Supplementary Fig. 5c ). This analysis uncovered a significant decrease in HAC1 nuclear signal intensity, mirrored by an increase in the cytoplasmic HAC1 mRNA signal, recapitulated by a significant decrease in the ratio of nuclear to cytoplasmic HAC1 mRNA signal intensity in isw1 Δ compared to WT cells (Fig. 4c ). This indicates that the absence of Isw1 correlates with a reduction of HAC1 mRNA steady-state nuclear localization. Similar results were observed when HAC1 mRNA localization was monitored after UPR induction or during UPR abatement (Supplementary Fig. 5c, d ). In a complementary approach, we used the measurement of transcripts co-immunoprecipitated with Cbp20, a subunit of the nuclear cap-binding protein, as a proxy for nuclear mRNA quantification. The amount of HAC1 transcripts co-immunoprecipitated with Cbp20 was significantly decreased in isw1 Δ compared to WT cells, further supporting that inactivation of ISW1 reduces the steady-state nuclear localization of the HAC1 transcript. A similar effect was observed for IOC2 , a previously defined Isw1 target, consistent with the reported nuclear mRNA retention activity of Isw1 [26] (Fig. 4d ). Altogether, our results demonstrated that Isw1 is required for the nuclear retention of HAC1 mRNA. Fig. 4: Isw1 is required for HAC1 mRNA nuclear retention. a Transcription shut-off experimental setting: Cells were treated with 2 mM DTT for 2 H. At t = 0, cells were washed and transcription was blocked by addition of 0.2 mg/mL phenanthroline in fresh media. Samples were collected for analysis at t = 0, 10’ and 20’. b The subcellular localization of the HAC1 transcript after blocking transcription with phenanthroline was analyzed in WT and isw1 Δ cells by FISH using Quasar®670 - HAC1 probes. White arrows point to transcription sites. Scale bar, 5 μm. For each time point, the percentage of cells showing a nuclear dot was scored. n = 3 independent experiments, mean ± s.d. Unpaired one-tail t -test ( p values relative to WT: 0.006583954 and 0.0194876 for10’ and 20’ respectively). c HAC1 mRNA subcellular localization was analyzed by FISH using Quasar®670- HAC1 probes. White arrows point to transcription sites. Red arrows highlight nuclei with high- intensity HAC1 mRNA signal (see also inset). Scale bar, 5 μm. Nuclear and cytoplasmic Quasar®670- HAC1 signal intensities were measured in at least 200 cells. Unpaired two-tailed t -test ( p values < 0.0001 for nuclear, cytoplasmic and nuclear/cytoplasmic signal intensities). Signal intensities were plotted into whiskers plots. Boxes extend from the 25th to 75th percentiles. The line in the middle of the box is plotted at the median. Whiskers are plotted down to the minimum and up to the maximum value, and each individual value is plotted as a point superimposed on the graph. Two independent biological replicates were performed with similar results. d The Cbp20- HAC1 / IOC2 mRNA interactions are reduced in isw1 Δ cells. RNA immunoprecipitation experiments (RIP) were performed with TAP-tagged Cbp20 WT and isw1 Δ cells. The ratio of co-immunoprecipitated HAC1 or IOC2 (Isw1 target) RNA to total RNA present in each strain relative to WT was quantified by qRT-PCR. Untagged WT cells were used as a negative control. n = 3 independent experiments, mean ± s.d. Unpaired one-tail t -test ( p values relative to WT Cpb20-Tap: Untagged: 1,0982E-05, isw1 Δ Cpb20-Tap: 6,55914E-05 for HAC1 ; p values relative to WT Cpb20-Tap: Untagged: 0,003149472, isw1 Δ Cpb20-Tap: 0,003733708 for IOC2 ). Full size image HAC1 IBM1 deletion phenocopies ISW1 inactivation To evaluate the influence of the Isw1- HAC1 mRNA interaction on the UPR, we sought to design a mutant version of HAC1 impaired for its ability to bind Isw1. The HAC1-3’ACT1 chimera (Fig. 1b ) could not be utilized for this purpose, due to its lack of a HAC1 ′s 3′UTR-located bipartite element (3′BE) which targets the transcript to Ire1 clusters for effective splicing [31] . We, therefore, determined the positions of Isw1 binding to the HAC1 transcript thanks to the CRAC data that had identified HAC1 as an Isw1 target transcript. These binding sites were clustered in two main regions within the 3′UTR of the HAC1 mRNA that we named IBM ( I sw1 B inding M otif) 1 and 2 (Fig. 5a ). We generated two mutants, hac1ΔIBM1 and hac1ΔIBM2 , deleted for the two Isw1 binding motifs located from either side of HAC1 ’s 3′BE (Fig. 5a ). Both mutants were more sensitive to Tm than WT cells (Fig. 5b, c Supplementary Fig. 6a ). However, hac1ΔIBM2 cells presented defective UPR activation (Supplementary Fig. 6b ), in line with their hypersensitivity to ER stress. This suggested that IBM2 deletion may perturb the structure of the 3’BE-containing stem and thus precluded further exploitation of this mutant. In contrast, HAC1 i was induced at similar levels in WT and hac1ΔIBM1 cells (Supplementary Fig. 6c compares WT and hac1ΔIBM1 ), indicating that IBM1 deletion did not significantly perturb the structure of the 3’BE. Isw1 RIP confirmed that deletion of HAC1 IBM1 significantly reduces the amount of HAC1 transcript co-immunoprecipitated with Isw1 (Fig. 5d ). Remarkably, deletion of IBM1 led to defective UPR attenuation (Fig. 5e and Supplementary Fig. 6c raw data), decreased steady-state HAC1 mRNA nuclear localization (Fig. 5f ), phenocopying ISW1 loss-of-function. In addition, IBM1 deletion was epistatic to inactivation of ISW1 (Fig. 5b, c, e, f , Supplementary Fig. 6c ), indicating that both mutations affect the same pathway. Finally, comparison of the UPR transcriptional output, the Tm sensitivity, and the subcellular localization of the HAC1 transcript in WT, isw1 ∆, hac1 Δ3’BE (Δ3’BE) and isw1 ∆, hac1 Δ3’BE cells reinforced the distinction between the 3’BE and the IBM regions. As previously reported, Δ3’BE cells were defective for HAC1 mRNA splicing and sensitive to ER stress [31] (Supplementary Fig. 6d, e ). They showed delayed HAC1 i production, presumably resulting from a compensatory increased expression of total HAC1 (Supplementary Fig. 6d ) and unperturbed HAC1 mRNA subcellular localization (Supplementary Fig. 6f ). Co-inactivation of ISW1 and the 3′BE resulted in increased levels of HAC1 Tot and prolonged HAC1 i expression, reduced HAC1 mRNA nuclear localization compared to WT and increased Tm sensitivity of the double mutant compared to each single mutant (Supplementary Fig. 6d–f ), implying that both mutations act in different processes. Taken together, these results indicate that the phenotype of isw1Δ cells is recapitulated by deletion of the HAC1 3’UTR-located IBM1 sequence, which is distinct from the 3′BE, and that mediates the interaction of the HAC1 transcript with Isw1. Fig. 5: Isw1 interacts with HAC1 mRNA 3′UTR. a Snapshot showing the positions of the deletions induced upon Isw1 cross-linking to HAC1 transcript. Isw1 CRAC experiments allow determining the positions to which a protein is crosslinked to an RNA target, owing to the errors generated by the reverse transcription reaction, that lead to deletions or mutations in the sequence reads, precisely at the sites of crosslink [27] , [68] . Red boxes indicate two major deletion sites in the 3’UTR of the HAC1 transcript named IBM1 and IBM2 (for I sw1 B inding M otif). b ISW1 and IBM1 deletions sensitize cells to Tm without showing additive effects. Fivefold serial dilutions of the indicated strains grown for 3 days at 30 °C with (+ER stress) or without (−ER stress) 0.6 μg/mL Tm. c Viability of the indicated strains was analyzed as described in Fig. 3b . n = 3 independent experiments, mean ± s.d. Unpaired one-tail t -tests ( p values relative to WT Untreated: 0.188927938, 0.188927938, 0.186383871, 0.190815197 for isw1 Δ, hac1 ΔIBM1, isw1Δhac1 ΔIBM1 and hac1 Δ respectively. p values relative to WT Tm: 5.19E−04, 1.29E−02, 8.60E−04 and 5.00227E−05 for isw1 Δ, hac1 ΔIBM1, isw1Δhac1 ΔIBM1 and hac1 Δ respectively. p value for hac1 ΔIBM1 isw1 Δ relative to isw1 Δ 1.99E−01. p value for hac1 ΔIBM1 isw1Δ relative to hac1 ΔIBM1 3.60E−03). d Deletion of HAC1 IBM1 domain reduces the amount of HAC1 transcript co-immunoprecipitated with Isw1. RIP experiments were performed in HTP tagged Isw1 cells expressing wild type HAC1 or hac1Δ IBM1 . Untagged WT cells were used as a negative control. The ratio of co-immunoprecipitated RNA to total relative to WT was quantified by qRT-PCR. n = 3 independent experiments, mean ± s.d. Unpaired one-tail t -tests ( p values relative to WT ( HAC1 , Isw1-HTP): 1.01E−04 and 3.14E−03 for Untagged and hac1 ΔIBM1, Isw1-HTP respectively for HAC1 target. p values relative to WT ( HAC1 , Isw1-HTP): 1.06396E−07 and 0.1510 for Untagged and hac1 ΔIBM1, Isw1-HTP respectively for IOC2 target). e hac1Δ IBM1 cells are defective for UPR termination. HAC1i relative to SCR1 mRNA expression during Tm UPR time courses, normalized to Tm 2H, as evaluated by qRT-PCR in the indicated strains. n = 4 independent experiments, mean ± s.d. Unpaired one-tail t-tests ( p values Wash 3H relative to Untreated: 3.67E-01, 7.25E-04, 4.96E-02 and 6.40E-04 for WT, isw1 Δ, hac1 ΔIBM1 and isw1Δhac1 ΔIBM1 strains respectively. p value Wash 3H isw1Δhac1 ΔIBM1 relative to isw1 Δ: 1.15E-01). Unnormalized data are shown in Supplementary Fig. 5c . f Deletion of IBM1 reduces the steady-state nuclear localization of HAC1 mRNA. HAC1 mRNA subcellular localization was analyzed by FISH using Quasar®670- HAC1 probes in the indicated strains. The nuclear to cytoplasmic ratio of HAC1 mRNA signal intensity was quantified. As in Fig. 4c , Nuclear and cytoplasmic Quasar®670- HAC1 signal intensities were measured in at least 200 cells. Unpaired two-tailed t -test ( p values < 0.0001 for isw1 Δ, hac1 ΔIBM1 and isw1Δhac1 ΔIBM1 strains relative to WT and for hac1 ΔIBM1 relative to isw1 Δ and to isw1Δhac1 ΔIBM1. p value 0.6402 for isw1Δhac1 ΔIBM 1relative to isw1 Δ). Nuclear to cytoplasmic ratio were plotted into whiskers plots. Boxes extend from the 25th to 75th percentiles. The line in the middle of the box is plotted at the median. Whiskers are plotted down to the minimum and up to the maximum value, and each individual value is plotted as a point superimposed on the graph. Two independent experiments were performed with similar results. Full size image Overexpression of Isw1 negatively regulates the UPR Since Isw1 can restrict cytoplasmic localization of transcripts, we wondered whether its overexpression could rescue mutants defective for UPR termination, by increasing HAC1 mRNA nuclear localization and thereby limiting its splicing. We therefore overexpressed Isw1 in WT or ire1D828A cells (Supplementary Fig. 7a ), which led to an increased steady-state nuclear localization of the HAC1 transcript (Supplementary Fig. 7b ). As reported, the growth and viability of ire1D828A cells upon Tm treatment was severely affected compared to WT (Fig. 6a, b ), which was associated with decreased but sustained HAC1 splicing upon 2-hour Tm induction and after wash-out of the drug respectively (Supplementary Fig. 7c, d ) indicating defective UPR termination. Remarkably, overexpression of Isw1 partially rescued the growth of ire1D828A cells in the presence of Tm, while it was slightly deleterious to the growth of WT cells (Fig. 6a, b ). Monitoring the transcriptional UPR output in these cells during Tm-induced UPR time-courses revealed that Isw1 overexpression correlated with a significant reduction of HAC1 splicing in WT—in line with a significant reduction of Hac1 expression (Supplementary Fig. 7e )—and ire1D828A cells (Fig. 6c, d ). In addition, in ire1D828A cells, this was associated with an improvement of the recovery of Pdi1’s glycosylation (Fig. 6e lanes 11, 12), suggesting a recovery of the ER oxidative protein folding capacity. In contrast, Isw1 overexpression marginally delayed Pdi1’s glycosylation recovery in WT cells (Fig. 6d , lanes 9, 10), which may result from the decrease in HAC1 mRNA splicing. Thus, Isw1 overexpression is able to influence the UPR, likely by limiting HAC1 splicing. Fig. 6: Isw1 overexpression negatively regulates the UPR. a Isw1 overexpression sensitizes WT cells to Tm but partially rescues the growth of ire1D828A cells on Tm. Fivefold serial dilutions of the indicated strains grown for 3 days at 30 °C on selective media containing (+ER stress) or not (−ER stress) 0,4 μg/mL Tm. b Viability of the indicated strains was analyzed as described in Fig. 3b . n = 3 independent experiments, mean ± sd. Unpaired one-tailed t -tests ( p values under Tm conditions: WT + p ADH ISW1 −2FL relative to WT: 1.28E−03, ire1D828A + p ADH ISW1 −2FL relative to ire1D828A: 5.67E−03). c , d Isw1 overexpression impairs HAC1 mRNA splicing. qRT-PCR analysis of the expression levels of HAC1 i, HAC1 u, and HAC1 Tot relative to WT in the indicated strains. n = 5 independent experiments, mean ± s.d. Unpaired one-tailed t -tests ( p values % HAC i for WT + p ADH ISW1 −2FL relative to WT: 3.23E−03, 5.78E−03, 3.62E−03 and 1.34E−03 for Untreated, Tm 2H, Wash 3H and Wash O/N conditions respectively. p values % HAC i for ire1D828A + p ADH ISW1 −2FL + p ADH ISW1 −2FL relative to ire1D828A : 3.25E−0, 8.76E−04, 1.27E−03 and 8.75E−04 for Untreated, Tm 2H, Wash 3H and Wash O/N conditions respectively). p values of HAC1 i, HAC1 u and HAC1 Tot are shown in the source data file. Unnormalized values shown in Supplementary Fig. 7b, c . e Isw1 overexpression improves Pdi1 re-glycosylation in ire1D828A cells during Tm UPR time course. Total protein extracts from WT and ire1D828A cells overexpressing or not Isw1 and collected during Tm UPR time courses were analyzed by western blot with anti-Pdi1 antibodies. *indicates the persistence of deglycosylated Pdi1. Three independent experiments were performed with similar results. Full size image ISW1 is itself induced by the UPR ISW1 was previously described in a genome-wide analysis as a UPR transcriptional target [11] , suggesting that UPR-mediated ISW1 induction could participate in a negative loop of UPR regulation. We verified the induction of ISW1 by ER stress (Fig. 7a, b ) and analyzed the effect of stress on the interaction of Isw1 with RNA using the RIP assay. ER stress increased the amount of mRNA co-immunoprecipitated with Isw1 (Fig. 7c ), supporting the possibility that this enhanced Isw1- HAC1 mRNA interaction could contribute to the attenuation phase of the UPR by limiting HAC1 mRNA nuclear export. Swapping of the ISW1 promoter region for that of IOC4 , a non-UPR target gene with a similar transcription rate [38] , prevented its ER stress induction (Fig. 7a, b ). Accordingly, cells unable to induce ISW1 in response to ER stress showed defective UPR attenuation as evaluated by monitoring HAC1i level during Tm-induced UPR time-course (Fig. 7d , Supplementary Fig. 8a , unnormalized) and a slight but consistent increase in sensitivity to tunicamycin (Fig. 7e, f ). Ultimately, our results support a model in which Isw1 stands as a novel actor of the UPR. ER stress-induced Isw1, through its ability to directly bind the 3’UTR of the HAC1 transcript, limits its nuclear export and therefore cytoplasmic splicing, allowing for a negative feed-back tuning of the UPR, necessary for its accurate termination (Fig. 7g ). Fig. 7: UPR-mediated ISW1 induction allows a negative feedback control of the pathway. a Swapping of ISW1 endogenous promoter prevents its ER stress induction. Tm-induced ISW1 expression is abolished in cells expressing p IOC4 ISW1 while KAR2 induction is unaffected, as evaluated by qRT-PCR analysis. n = 3 independent experiments, mean ± s.d. Unpaired one-tailed t -tests ( p values relative to Untreated for ISW1 target: 4.22E−03 and 3.83E−01 for isw1Δ +p ISW1 −2FL and isw1Δ +p IOC4 ISW1 −2FL respectively. p values relative to Untreated for KAR2 target: 6.94E−04 and 1.70E−07 for isw1Δ +p ISW1 −2FL and isw1Δ +p IOC4 ISW1 −2FL respectively). b Swapping of ISW1 endogenous promoter prevents the induction of Isw1 by Tm. Total protein extracts from isw1Δ cells expressing pISW1-2FL or isw1Δ+p IOC4 ISW1-2FL grown in the presence (+) or absence (−) of 1 μg/mL Tm for 2 H were analyzed by western blot with anti-FLAG, anti-Pab1 (loading) and anti-Kar2 (UPR induction) antibodies and the level of Isw1 relative to Pab1 was quantified. n = 3 independent experiments, mean ± s.d. Unpaired one-tailed t -tests ( p values Tm 2 H relative to Untreated: 2.69E−02 and 4.96E−01 for isw1Δ + pISW1-2FL and isw1Δ+p IOC4 ISW1-2FL cells respectively). c The interaction between Isw1 and its mRNA targets is fostered by ER stress. RIP assays in Isw1-HTP cells treated or not with 2 mM DTT for 1 H. Ratio of co-immunoprecipitated RNA to total RNA relative to untreated quantified by qRT-PCR. n = 3 independent experiments, mean ± s.d. Unpaired one-tailed t -tests ( p values relative to Untreated for HAC1 target: 2.77E−03 and 1.12E−03 for Untagged and Isw1-HTP + DTT respectively. ( p values relative to Untreated for IOC2 target: 3.21E−05 and 1.18E−02 Untagged and Isw1-HTP + DTT respectively. p values relative to Untagged for HAC1 target: 2.77E−03 and 5.65E−04 for Isw1-HTP, Untreated and Isw1-HTP + DTT respectively. p values relative to Untagged for IOC2 target: 3.21412E−05 and 9.68E−04 for Isw1-HTP, Untreated and Isw1-HTP + DTT respectively). d Cells expressing non-UPR-inducible ISW1 (p IOC4 ISW1 ) are defective for UPR termination. HAC1i normalized to SCR1 mRNA expression during Tm UPR time courses, relative to Tm 2 H, as evaluated by qRT-PCR in isw1Δ cells expressing pISW1 or isw1Δ+p IOC4 ISW1 . n = 3 independent experiments, mean ± s.d. Unpaired one-tailed t -tests ( p values Wash 3 H relative to Untreated: 1.10E−01and 2.56E−03 for isw1Δ + pISW1-2FL and isw1Δ+p IOC4 ISW1-2FL cells respectively. Unnormalized values shown in Supplementary Data Fig. 8a . e Cells deficient for UPR-mediated ISW1 induction are more sensitive to Tm than WT. Fivefold serial dilutions of the indicated strains grown in the presence (+ER stress) or absence (−ER stress) of 0.4 μg/mL Tm. f Viability of the indicated strains was analyzed as described in Fig. 3b . n = 3 independent experiments, mean ± s.d. Unpaired one-tailed t -tests ( p values relative to WT under Untreated conditions: 4.46E−01, 5.25E−02 and 3.31E−01 for isw1Δ , p IOC4 ISW1 and ire1Δ cells respectively. p values relative to WT under Tm conditions: 5.19E−04, 6.18E−03 and 3.11E−04 for isw1Δ , p IOC4 ISW1 and ire1Δ cells respectively). g Model: Cross-talk between Isw1-mediated nuclear mRNA quality control and the Unfolded protein response. The nuclear export of HAC1 mRNA is restricted by direct binding of the chromatin remodeler Isw1 to its 3′UTR. This nuclear retention activity of Isw1 is reinforced by its UPR induction and appears critical for accurate UPR termination and cell survival upon ER stress. Full size image We previously reported that the chromatin remodeler Isw1, although deprived of canonical RNA binding domains, “moonlights” as an RNA binding protein (RBP) that prevents untimely nuclear export of maturing or improper mRNAs. In the present study, we underscore a case of molecular cross-talk between this newly evidenced mRNA quality control pathway and the evolutionarily conserved UPR whose activation strictly relies on the cytoplasmic splicing of the Hac1 encoding mRNA. We show that the direct binding of Isw1 to the 3′UTR of HAC1 mRNA allows precise controlling of its nuclear export, and therefore of its translation and of UPR signaling. ISW1 being itself an UPR target gene, we propose that ER stress-induced Isw1 is a key effector of the negative feedback loop that abates UPR signaling. Our CRAC experiment demonstrates, as previously reported [26] , the binding of Isw1 to multiple mRNA species whose nuclear export are expected to be limited by Isw1. While we cannot exclude that these putative Isw1 targets might also impact UPR signaling, we assume that Isw1 binding to HAC1 mRNA has stronger physiological consequences because it not only regulates the level of the transcript in the cytoplasm but also affects its splicing and thereby the synthesis of the short-lived Hac1 protein. Although the effect of ISW1 inactivation on UPR signaling may seem modest, it stands in a similar range to that of previous reports. As such, inactivation of PDIA6, a protein disulfide isomerase that limits UPR signaling, resulted in increased XBP1 splicing during UPR abatement, accompanied with increased sensitivity to ER stress [39] . While in agreement with the literature, it is currently unclear why, in isw1Δ cells, deficient UPR abatement leads to incomplete stress mitigation and decreased cell viability upon ER stress [3] , [4] , [13] , although UPR induction appears indistinguishable from WT cells. An appealing explanation is that sustained UPR activation overloads the translocation machinery [4] , [40] , leading to mislocalization of ER resident proteins, some of which having crucial functions in ER homeostasis. This is supported by our Pdi1 glycosylation time-courses. Upon Tm wash, inhibition of protein glycosylation is released and coincides with the appearance of five discrete bands above deglycosylated Pdi1. These likely correspond to the mono, di, tri, tetra and penta glycosylated forms of the protein that is translocated post-translationally [41] and would receive the N-glycan on each of its consensus Asn residue, as it emerges into the ER lumen. The delayed Pdi1 glycosylation observed in isw1 Δ cells would thus be symptomatic of a saturation of the translocation apparatus that can virtually concern a wide-range of ER-destined proteins, ultimately leading to increased sensitivity to ER stress. Alternatively, this could result from the activation of cell death pathway(s) triggered upon persistent Ire1/Hac1 signaling. This would be reminiscent of mammals where the UPR initially engages adaptive outputs to lessen the load of unfolded proteins, but which, under chronic or unresolved ER stress causes cells commitment to apoptosis [2] . ISWI factors were previously implicated in the regulation of stress responses. Yeast Isw1, in combination with other chromatin remodelers, has been associated with the regulation of expression of heat stress genes [42] , [43] . Similarly, homologs of Isw1 were reported to contribute to stress-induced memory of heat shock genes in plants [44] or to control the expression of cytosolic chaperones in response to mitochondrial stress in C. elegans [45] . In all these circumstances however, the influence of ISWI on the stress responses are mediated by a transcriptional effect whereas the Isw1-mediated UPR regulation that we report relies on its RNA binding activity. Strikingly, the subcellular localization of HAC1 mRNA proves to be crucial for accurate UPR signaling. Seminal work from Peter Walter’s laboratory demonstrated that a 3′BE contained in HAC1 3′UTR is essential to its targeting to Ire1 foci [31] . Our data unveil that the 3′UTR carries additional localization signals: the IBM1 motif, whose interaction with Isw1 allows fine-tuning the rate of HAC1 transcript export to the cytoplasm. Given the previously reported low basal activity of Ire1 [46] , [47] , this nuclear export control appears essential to prevent excessive or untimely HAC1 mRNA splicing, as observed in isw1 Δ cells in the absence of stress (Fig. 2b, c and ref. 46 . The ability of overexpressed Isw1 to shape the UPR, and especially to rescue the phenotypes of ire1D828A cells, shores up the critical function of the Isw1-mediated HAC1 mRNA retention in accurate UPR attenuation and is lending support to the prominent role of mRNA nuclear retention on the regulation of gene expression. With respect to the UPR, this activity of Isw1 is remarkable for it highlights a previously unrecognized level of regulation of the signaling abatement, that emanates from the nucleus and acts synergistically with the previously described Ire1 deactivation-mediated pathways of UPR attenuation. Although poly(A) RNA nuclear retention was acknowledged more than 40 years ago [48] , its potential significance for gene expression has long been ignored. It drew growing attention over the last decade and was shown to serve various functions [49] , [50] , such as quality control, rapid adaptation to stress, regulation of protein level, or more recently to provide a general mean to buffer “noisy” gene expression resulting from bursts in gene transcription [51] , [52] . Because HAC1 mRNA is exported from the nucleus in WT conditions, its interaction with Isw1 is expected to be weak or transient and outcompeted by the binding of nuclear export factors, therefore only “putting a break” on the kinetics of its nuclear export. While we observed an increase in the Isw1- HAC1 mRNA interaction upon ER stress due to ISW1 UPR induction, it is unknown whether the affinity of Isw1 for RNA is regulated upon specific conditions. Given the prominence of the intensity and duration of the UPR for cell fate decisions under ER stress, ISWI/SMARCA5, whose RNA binding activity is conserved in Drosophila [53] and mammalian cells [54] , [55] , appears as a promising target for therapeutic intervention against the growing number of human diseases associated with ER stress and inappropriate UPR regulation [56] , [57] . Interestingly, GWA studies associated a SNP yielding a truncated mutant of human SMARCA5 to Amyotrophic lateral sclerosis [58] , a disease with multiple connections to ER stress and RNA metabolism [59] , [60] . Yeast strains All experiments were performed using Saccharomyces cerevisiae strains of the W303 background. Strains were grown at 30 °C according to classical procedures in standard yeast extract peptone dextrose (YPD) or dropout base supplemented with the appropriate CSM-amino acid (MP Biomedicals, LCC) media. To induce ER stress, yeast cells were treated with 2 mM of dithiothreitol (DTT, VWR) or 1 μg/ml of tunicamycin (Tm, Sigma). Gene deletions and tagging were created by one-step PCR mediated strategy, as described in ref. 61 . The HAC1- 3′UTR ACT1 chimeric strain was built by insertion of a KanMx cassette 283 bp downstream of ACT1 , followed by PCR amplification of a 3′UTR ACT1 -KanMx product flanked by 50 bp sequences surrounding HAC1 3′UTR, that was transformed into the WT strain for replacement of the endogenous HAC1 3′UTR. IBM1 (positions 39–135 of HAC1 3′UTR) and IBM2 (300–428) deletions were generated by mutagenesis (Q5® Site directed mutagenesis, NEB) in pRS316- HAC1 and introduced genomically by PCR with a KanMx cassette. All mutations were verified by sequencing. 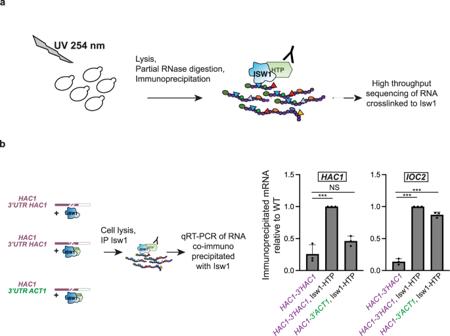Fig. 1: Isw1 interacts with the 3’UTR ofHAC1mRNA. aScheme depicting the identification of Isw1-bound transcripts by in vivo UV-crosslinking and analysis of cDNA. Growing yeast cells expressing dual affinity tagged (HIS6-TEV-PrA) Isw1 were UV-irradiated with 254 nm UV light to covalently crosslink RNA-protein complexes, which were immunopurified under stringent wash condition to prevent the recovery of indirect RNA targets. After ligation of linkers, crosslinked RNAs were converted to cDNA, PCR amplified, and sequenced.bThe interaction betweenHAC1mRNA and Isw1 is mediated by its 3′UTR. RIP assays were performed with HTP tagged Isw1 in cells expressing wild typeHAC1(HAC13′UTRHAC1) or a chimericHAC1(HAC13′UTRACT1). Untagged WT cells were used as a negative control. The ratio of co-immunoprecipitatedHAC1orIOC2RNA to total RNA relative to WT was quantified by qRT-PCR.n= 3 independent experiments, mean ± s.d. Unpaired one-tailt-test (pvalues relative to No Tag:HAC1, Isw1-HTP: 4.56E−04HAC1-3′ACT1, Isw1-HTP: 9.95E−02 forHAC1and Isw1-HTP: 2.89693E−06,HAC1-3′ACT, Isw1-HTP: 3.55186E−05 forIOC2). Yeast cells used in this study are described in Supplementary Table 1 . Plasmids pRS416 IOC4 - ISW1-2FL plasmid was built by replacing the endogenous ISW1 promoter in plasmid pRS416- ISW1-2FL by the IOC4 promoter (603 bp region upstream of ATG) amplified from WT W303 strain, via homologous recombination. The plasmids were verified by sequencing. 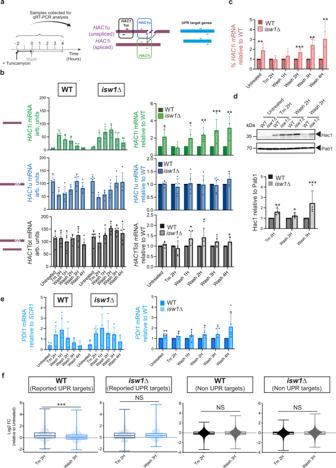Fig. 2:ISW1inactivation prevents accurate UPR termination. aTm UPR time course experimental setting: WT andisw1Δ exponentially growing cells were treated with 1 μg/mL tunicamycin for 2 h, washed and resuspended in Tm free medium. Samples were collected att= −2 h (Untreated),t= 0 (Tm 2 H),t= 1 h (Wash 1 H),t= 2 h (Wash 2 H),t= 3 h (Wash 3 H), andt= 4 h (Wash 4 H) for analysis ofHAC1mRNA splicing and expression of UPR target genes by qRT-PCR using the depicted primers.bqRT-PCR analysis of the expression levels ofHAC1i,HAC1u, andHAC1Tot relative toSCR1or to WT, in WT andisw1Δ cells during the Tm UPR time course depicted inb.n= 5 independent experiments, mean ± s.d.cHAC1splicing is sustained inisw1Δ compared to WT cells during Tm UPR time course. The percentage of splicedHAC1(HAC1i /HAC1Tot x100) was calculated from the values obtained inb.n= 5 independent experiments, mean ±  s.d. Unpaired one-tailt-test (pvalues relative to WT: 4.20E−03 4.40E−01, 8.67E−02, 1.04E-03, 2.45E−03, 1.14E−02 for Untreated, Tm 2 H, Wash 1 H, Wash 2 H, Wash 3 H, Wash 4 H respectively).dHac1 expression is sustained inisw1Δ compared to WT cells. Total protein extracts from WT andisw1Δ cells treated or not with 1 μg/mL Tm for 2 H were analyzed by western blot with anti-Hac1 and Pab1 (loading) antibodies. The level of Hac1 and Pab1 was quantified.n= 4 independent experiments, mean ± s.d. Unpaired one-tailedt-test (pvalues relative to WT: 0.004387283, 0.039668848, 0.024072787 at Tm 2 H, Wash 2 H, Wash 3 H respectively).eThe mRNA expression level of canonical Hac1 targets is prolonged inisw1Δ cells compared to WT, as evaluated by qRT-PCR analysis ofPDI1transcript expression relative toSCR1during Tm UPR time courses.n= 5 independent experiments, mean ± s.d.fWhisker plots of expression fold change (Log2 FC) for all UPR (defined in ref.11) and non-UPR target genes at Tm 2 H and Wash 3 H relative to untreated in WT andisw1Δ cells. Boxes extend from the 25th to 75th percentiles. The line in the middle of the box is plotted at the median. Whiskers are plotted down to the minimum and up to the maximum value, and each individual value is plotted as a point superimposed on the graph.n= 3 independent biological replicates. Paired two-tailedt-test (pvalues for WT UPR targets <0.00001, forisw1Δ UPR targets 0.1408, for WT non-UPR targets 0.053, forisw1Δ non-UPR targets 0.1048). Plasmids used in this study are described in Supplementary Table 2 . Plate-based growth assays Cells inoculated in the appropriate medium and grown overnight at 30 °C were diluted to OD 600 = 0.4 grown for 2 h and re-diluted to OD 600 = 0.8 in water. Fivefold serial dilutions were plated with a Replica plater. Plates were imaged after 3 days of growth at 30 °C. When indicated, tunicamycin was added to the growth medium at concentrations ranging from 0.2 to 0.8  μg/mL. Control plates contained 4 μL of DMSO (drug carrier). Each presented growth assay is a representative example of at least three biological replicates. Viability assay Cells were suspended in PBS and stained with 5 μg/mL propidium iodide (1 mg/mL stock solution, dissolved in water) for 20 min in the dark at room temperature. PI fluorescence was examined from at least 400 cells in three biological replicates under a fluorescence microscope and red fluorescent cells (dead) were counted. Chromatin immunoprecipitation Cells were cross-linked in the presence of 1% formaldehyde for 10 min at 25 °C. After quenching with 100 mM glycine and washing with Tris-buffered saline, cell pellets were resuspended in 1 ml lysis buffer (50 mM Hepes pH 7.5, 140 mM NaCl, 1 mM EDTA, 1% triton X-100, 0.1% deoxycholate, 1X protease inhibitors cocktail, complete EDTA-free, Roche) and lysis was achieved in the presence of acid washed glass beads (Sigma) using the MagNAlyser (Roche). Cell lysates were collected and sonicated using a Bioruptor (Diagenode) to shear DNA for three runs of 10 min. Solubilized chromatin was retrieved through a 5 min-centrifugation at 2500 × g . Anti-RNA Polymerase II antibodies (OptimAb™ RNA Polymerase II 8WG16, Eurogentec) were added and immunoprecipitation was performed by overnight rotation at 4 °C. Protein-G sepharose beads (GE Healthcare) were added to the samples for two additional hours. Washes were as follow: twice with lysis buffer, twice with lysis buffer containing 360 mM NaCl; twice with 10 mM Tris pH 8, 250 mM LiCl, 0.5% Nonidet-P40, 0.5% deoxycholate, 1 mM EDTA and once with 10 mM Tris–HCl pH 8, 1 mM EDTA. Elution was performed through a 20-min incubation at 65 °C in the presence of 50 mM Tris pH 8, 10 mM EDTA, 1% SDS. The eluate was deproteinized with proteinase K (Sigma, 0.2 mg/mL) and uncrosslinked for 30 min at 65 °C. Immunoprecipitated DNA was purified with the Qiaquick PCR purification kit (Qiagen) and quantified by real-time PCR with a QuantStudio5™ (Applied Biosystems™) according to the manufacturer’s instructions. qRT-PCR analysis and RNA immunoprecipitation For qRT-PCR analysis, RNA was isolated from 10 OD of exponentially growing cells washed in MilliQ water and snap frozen. RNA was extracted with the Nucleospin RNA II Kit (Macherey-Nagel), and reverse transcribed using the SuperScript II reverse transcriptase (Invitrogen). cDNA was quantified by qPCR (Master Mix PCR Power SYBR™ Green ThermoFisher; QuantStudio5™; Applied Biosystems™). Analysis of HAC1 mRNA splicing was performed as follows. Primers qAB 88/qAB91, qAB135/91 and qAB124/125 were designed to specifically amplify HAC1 u, HAC1 i and HAC1 Tot respectively, with qAB88 spanning the exon1-intron junction and qAB135 spanning the exon-exon junction of the transcript. Specificity of primers qAB88 and qAB135 was validated by qRT-PCR analysis performed on a mix of two plasmids bearing the u nspliced and s pliced form of HAC1 with the following ratios: u/s = 1/0-0.75/0.25-0.5/0.5- 0.25/0.75-0/1. The percentage of HAC1 mRNA splicing was assessed using the LEM-PCR method [62] . For the three amplicons ( HAC1 u, i, Tot), standard curves were generated from the same cDNA derived from the WT Tm 2H samples. The relative abundance of HAC1 u, HAC1 i and HAC1 Tot were used to derive two linear equations: 
    Untreated:x.HAC1u_Untreated=y.HAC1i_Untreated+HAC1Tot_Untreated
 (1) 
    Tm2H:x.HAC1u_Tm2H=y.HAC1i_Tm2H+HAC1Tot_Tm2H
 (2) The x and y values determined by solving these equations were substituted into the equation for each sample and allowed to determine the percentage of spliced HAC1 during UPR time-courses. RNA immunoprecipitations were performed from 2 g of frozen cell grindates prepared as previously described [26] . Immunoprecipitated RNA was isolated from proteins by treating samples with 40 μg Proteinase K (Roche) and 0.1% SDS for 30 min at 30 °C. RNA was extracted with the Nucleospin RNA II Kit (Macherey-Nagel), and reverse transcribed using the SuperScript II reverse transcriptase (Invitrogen). cDNA was quantified by qPCR as previously described. 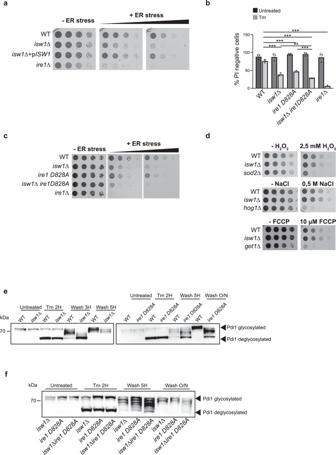Fig. 3:ISW1inactivated cells are sensitive to ER stress and defective for ER homeostasis reset. aisw1Δ cells are more sensitive than WT to tunicamycin: fivefold serial dilutions of the indicated strains grown for 3 days at 30 °C on selective media containing (+ER stress) or not (−ER stress) 0.4 μg/mL or 0.6 μg/mL Tm.bViability assay. Exponentially growing cells were treated or not with 1 μg/mL Tm for 24 H and stained with propidium iodide (PI). The percentage of PI negative cells is plotted. A minimum of 300 cells per condition were counted.n= 3 independent experiments, mean ± s.d. Unpaired one-tailt-test (pvalues relative to WT Untreated: 0.445937983, 0.093299173, 0.110093567, 0.41523827 forisw1Δ,ire1D828A, isw1Δire1D828Aandire1Δ respectively.pvalues relative to WT Tm: 0.000201098, 0.000243914, 2.46522E-05, 7.60488E-06 forisw1Δ,ire1D828A, isw1Δire1D828Aandire1Δ respectively.pvalue forire1D828A isw1Δ relative toisw1Δ 0.00662224.pvalue forire1D828A isw1Δ relative toire1D828A5.76554E-05.cisw1Δ andire1D828Amutations have compounding effects. Fivefold serial dilutions of the indicated strains grown for 3 days at 30 °C on selective media containing (+ER stress) or not (−ER stress) 0.4 μg/mL or 0.6 μg/mL Tm.disw1Δ cells are not more sensitive than WT cells to oxidative, osmotic and mitochondrial stresses. Fivefold serial dilutions of the indicated strains grown for 2 days at 30 °C with or without 2.5 mM H2O2, 0.5 M NaCl or 10 μM Carbonyl cyanide-p-trifluoromethoxyphenylhydrazone (FCCP), a potent uncoupler of mitochondrial oxidative phosphorylation.sod2Δ,hog1Δ andget1Δ mutants respectively serve as positive controls for the effect of the stresses.e,fPdi1 re-glycosylation during Tm UPR time course. Total protein extracts from WT,isw1Δ,ire1D828A,andisw1Δire1D828Acells collected during Tm UPR time courses were analyzed by western blot with anti-Pdi1 antibodies. Three independent experiments were performed with similar results. Primers used in this study are described in Supplementary Table 3 . Deep sequencing mRNA sequencing libraries were prepared from polyA+ RNAs purified from 1μg of total RNA using NEBNext® UltraTM RNA Library Prep Kit for Illumina® (NEB, USA) following the manufacturer’s recommendations. A 150 bp read sequencing was Illumina sequenced with multiplexing. A mean of 17.7 ± 2.4 million passing Illumina quality filter reads was obtained for each of the samples. Library preparation and sequencing with Illumina technology were performed by Novogene (Novogene Co., Ltd). CRAC assay CRAC has been performed according to ref. 63 with the modifications described in ref. 64 . Briefly, 2 L of yeast cells expressing Isw1-HTP tag or Rpb-HTP tag were grown at 30 °C to OD 600 = 0.6 in CSM-Trp medium. Cells were UV crosslinked using a W5 UV crosslinking unit (UVO3 Ltd) for 50 s, harvested by centrifugation, washed in cold PBS and resuspended in TN150 buffer (50 mM Tris pH 7.8, 150 mM NaCl, 0.1% NP-40 and 5 mM β-mercaptoethanol, 2.4 mL/g of cells) supplemented with protease inhibitors (Complete, EDTA-free Protease Inhibitor Cocktail). The suspension was flash frozen in droplets and cells were mechanically broken with a Mixer Mill MM 400. Extracts were treated for one hour at 25 °C with DNase I (165 U/g of cells) to solubilize chromatin and clarified by centrifugation. Complexes were purified by a two-step procedure, the second one under denaturing conditions. Both purification steps were performed under high stringency (1 M NaCl). The protein fractionation step was performed with a Gel Elution Liquid Fraction Entrapment Electrophoresis (GelFree) system (Expedeon). Isw1-containing fractions were treated with 100 mg of proteinase K. RNAs were purified and reverse transcribed with Superscript IV (Invitrogen). The concentration of cDNAs in the reaction was estimated by quantitative PCR and accordingly PCR amplified. After treatment with 200 U/ml of Exonuclease I (NEB), DNA was purified using NucleoSpin Gel and PCR Clean-up (Macherey-Nagel) and sequenced using Illumina technology. Next-generation sequence analysis For RNA-Seq analysis, raw data were processed through in-house scripts. Paired-end clean reads were mapped to the reference genome using HISAT2 software. Reads were aligned to the S. cerevisiae reference genome (SaCer3). HTSeq software was used to analyze the gene expression levels in this experiment, using the union mode. Differential expression analysis between two conditions (three biological replicates per condition) was performed using DESeq2, R package. The resulting P values were adjusted using the Benjamini and Hochberg’s approach for controlling the false discovery rate (FDR). Genes with an adjusted P value < 0.05 found by DESeq2 were assigned as differentially expressed. CRAC datasets were analyzed as described [28] . The pyCRAC script pyFastqDuplicateRemover was used to collapse PCR duplicates using a 6 nucleotides random tag included in the 3’ adaptor. The resulting sequences were reverse complemented with Fastx reverse complement (part of the fastx toolkit, http://hannonlab.cshl.edu/fastx_toolkit/ ) and mapped to the R64 genome [65] with bowtie2 (−N 1) [66] . In order to identify with higher precision the binding position a further analysis was performed to extract deletions and mismatches inside the mapped reads and collect their positions in a coverage file. This step was performed with the peakCcall repository [64] . Protein extracts and immunoblotting Cells grown in the appropriate medium to OD 600 0.4 were treated with 1 μg/ml of Tm for 2 h when indicated. 20% trichloroacetic acid (TCA, Sigma) was added to the culture. 10 OD of cells were collected for each point, pelleted and washed in 20% TCA at 4 °C. Pellets were snap frozen in liquid nitrogen and further processed by cells resuspension in 200 μl of TCA 20% and disruption by vortexing for 10 mn at 4 °C in the presence of 100 μl of acid washed glass beads (Sigma). After beads removal, samples were centrifuged at 11,000 × g for 10 min and pellets were resuspended in Laemmli buffer, heated for 5 min at 95 °C. Protein were separated by SDS-PAGE and transferred onto a nitrocellulose membrane that was probed with the relevant antibody. Protein were detected by chemiluminescence (SuperSignal™ West Pico/Femto Chemiluminescent Substrate, ThermoFisher) and images were captured with the FUSION FX imaging system (Vilber). 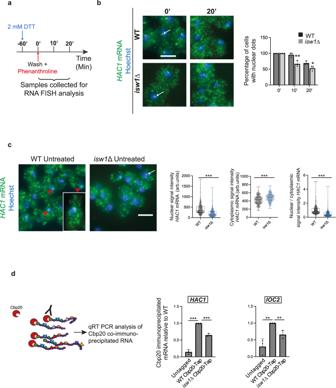Fig. 4: Isw1 is required forHAC1mRNA nuclear retention. aTranscription shut-off experimental setting: Cells were treated with 2 mM DTT for 2 H. Att= 0, cells were washed and transcription was blocked by addition of 0.2 mg/mL phenanthroline in fresh media. Samples were collected for analysis att= 0, 10’ and 20’.bThe subcellular localization of theHAC1transcript after blocking transcription with phenanthroline was analyzed in WT andisw1Δ cells by FISH using Quasar®670 -HAC1probes. White arrows point to transcription sites. Scale bar, 5 μm. For each time point, the percentage of cells showing a nuclear dot was scored.n= 3 independent experiments, mean ± s.d. Unpaired one-tailt-test (pvalues relative to WT: 0.006583954 and 0.0194876 for10’ and 20’ respectively).cHAC1mRNA subcellular localization was analyzed by FISH using Quasar®670-HAC1probes. White arrows point to transcription sites. Red arrows highlight nuclei with high- intensityHAC1mRNA signal (see also inset). Scale bar, 5 μm. Nuclear and cytoplasmic Quasar®670-HAC1signal intensities were measured in at least 200 cells. Unpaired two-tailedt-test (pvalues < 0.0001 for nuclear, cytoplasmic and nuclear/cytoplasmic signal intensities). Signal intensities were plotted into whiskers plots. Boxes extend from the 25th to 75th percentiles. The line in the middle of the box is plotted at the median. Whiskers are plotted down to the minimum and up to the maximum value, and each individual value is plotted as a point superimposed on the graph. Two independent biological replicates were performed with similar results.dThe Cbp20-HAC1/IOC2mRNA interactions are reduced inisw1Δ cells. RNA immunoprecipitation experiments (RIP) were performed with TAP-tagged Cbp20 WT andisw1Δ cells. The ratio of co-immunoprecipitatedHAC1orIOC2(Isw1 target) RNA to total RNA present in each strain relative to WT was quantified by qRT-PCR. Untagged WT cells were used as a negative control.n= 3 independent experiments, mean ± s.d. Unpaired one-tailt-test (pvalues relative to WT Cpb20-Tap: Untagged: 1,0982E-05,isw1Δ Cpb20-Tap: 6,55914E-05 forHAC1;pvalues relative to WT Cpb20-Tap: Untagged: 0,003149472,isw1Δ Cpb20-Tap: 0,003733708 forIOC2). Antibodies used in this study are described in Supplementary Table 4 . Fluorescence in situ hybridization FISH was performed as previously described [26] , [67] with minor modifications. Cells grown in the appropriate media were fixed by adding parafolmaldehyde to the media at the final concentration of 4%. Fixation was performed for 45 min at room temperature (RT) on a rotating wheel. After 2 washes in wash buffer (100 mM KHPO4, pH 7.5), cells were pelleted and resuspended in spheroplast buffer (1.2 M sorbitol, 100 mM KHPO 4 , pH 7.5) supplemented with 0,5 mg/mL 100 T zymolyase and 2 mM vanadyl-ribonucleoside complex. Digestion was performed for approximately 15 min at 30 °C (until cell wall digestion of >80% of the cells). Spheroplasts were carefully washed twice in cold spheroplast buffer, resuspended in 70% ethanol and stored for at least 12 h at 4 °C. After cell rehydratation by resuspension in spheroplast buffer for 15 min at RT, spheroplasts were hybridized in hybridization buffer (Formamide 50%, Dextrane sulfate 10%, 4X SSC, 1X Denhardts, 125 mg/ml E. coli tRNA, 500 mg/ml salmon sperm DNA) supplemented with 2 ng of HAC1 -Quasar 670 probes and 2 mM vanadyl-ribonucleoside for 12 h in the dark at 30 °C. The next day, spheroplasts were washed twice in 2XSSC at 30 °C for one hour and 1XSSC for 30 min at room. DNA was stained with Hoechst 33342 (Sigma) and spheroplasts mounted onto mounting media. All coverslips were finally washed in 1XPBS plus Hoechst and mounted onto Vectashield© antifade mounting media. The HAC1 FISH probe was purchased from Biosearch technologies and contains a blend of 27 oligos spanning HAC1 exons labeled with Quasar®670. Probe specificity was verified against a hac1∆ strain. Quantifications were performed on maximum intensitiy z projections. For quantification of nuclear signal intensities, nuclei were segmented from the Hoechst images, the overlapping HAC1 Quasar®670 signals were determined using the “image calculator” function of the ImageJ software and measured with the “Analyze particles” function. Cytoplasmic signal intensities were measured in the same cells from random cytoplasmic circular ROI (1 μm radius). Fluorescence microscopy Three-dimensional stacks with a 0.2-μm step were acquired by 3D deconvolution microscopy using a Axiovert 200 M microscope (Carl Zeiss MicroImaging, Inc.) with a 63X oil immersion objective (NA = 1.4). Images were captured using a monochrome digital camera (Axiocam MRm; Carl Zeiss MicroImaging, Inc). Maximum intensity projections were performed using ImageJ software. Statistics and reproducibility Every depicted blot or growth assay is representative of at least three independent and reproducible experiments. Plots and statistical analysis were performed using Excel (Microsoft) for qRT-PCR analysis or Prism (Graphpad) for RNAseq analysis and RNA FISH quantification. Statistic tests and p values are described in the figure legends. Significance of the observed differences (* p value 0.01–0.05; ** p value 0.001–0.01; *** p value <0.001). For each experiment, the value of every data point as well as p values are provided in the source data file. 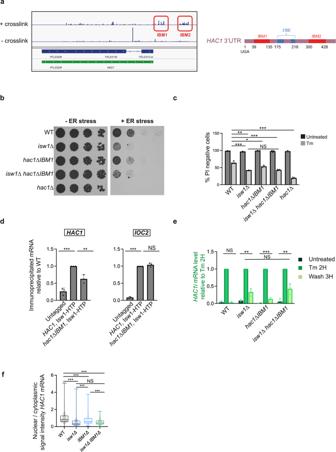Fig. 5: Isw1 interacts withHAC1mRNA 3′UTR. aSnapshot showing the positions of the deletions induced upon Isw1 cross-linking toHAC1transcript. Isw1 CRAC experiments allow determining the positions to which a protein is crosslinked to an RNA target, owing to the errors generated by the reverse transcription reaction, that lead to deletions or mutations in the sequence reads, precisely at the sites of crosslink27,68. Red boxes indicate two major deletion sites in the 3’UTR of theHAC1transcript named IBM1 and IBM2 (forIsw1BindingMotif).bISW1and IBM1 deletions sensitize cells to Tm without showing additive effects. Fivefold serial dilutions of the indicated strains grown for 3 days at 30 °C with (+ER stress) or without (−ER stress) 0.6 μg/mL Tm.cViability of the indicated strains was analyzed as described in Fig.3b.n= 3 independent experiments, mean ± s.d. Unpaired one-tailt-tests (pvalues relative to WT Untreated: 0.188927938, 0.188927938, 0.186383871, 0.190815197 forisw1Δ,hac1ΔIBM1,isw1Δhac1ΔIBM1 andhac1Δ respectively.pvalues relative to WT Tm: 5.19E−04, 1.29E−02, 8.60E−04 and 5.00227E−05 forisw1Δ,hac1ΔIBM1,isw1Δhac1ΔIBM1 andhac1Δ respectively.pvalue forhac1ΔIBM1isw1Δ relative toisw1Δ 1.99E−01.pvalue forhac1ΔIBM1isw1Δrelative tohac1ΔIBM1 3.60E−03).dDeletion ofHAC1IBM1 domain reduces the amount ofHAC1transcript co-immunoprecipitated with Isw1. RIP experiments were performed in HTP tagged Isw1 cells expressing wild typeHAC1orhac1Δ IBM1. Untagged WT cells were used as a negative control. The ratio of co-immunoprecipitated RNA to total relative to WT was quantified by qRT-PCR.n= 3 independent experiments, mean ± s.d. Unpaired one-tailt-tests (pvalues relative to WT (HAC1, Isw1-HTP): 1.01E−04 and 3.14E−03 for Untagged andhac1ΔIBM1, Isw1-HTP respectively forHAC1target.pvalues relative to WT (HAC1, Isw1-HTP): 1.06396E−07 and 0.1510 for Untagged andhac1ΔIBM1, Isw1-HTP respectively forIOC2target).ehac1Δ IBM1cells are defective for UPR termination.HAC1irelative toSCR1mRNA expression during Tm UPR time courses, normalized to Tm 2H, as evaluated by qRT-PCR in the indicated strains.n= 4 independent experiments, mean ± s.d. Unpaired one-tail t-tests (pvalues Wash 3H relative to Untreated: 3.67E-01, 7.25E-04, 4.96E-02 and 6.40E-04 for WT,isw1Δ,hac1ΔIBM1 andisw1Δhac1ΔIBM1 strains respectively.pvalue Wash 3Hisw1Δhac1ΔIBM1 relative toisw1Δ: 1.15E-01). Unnormalized data are shown in Supplementary Fig.5c.fDeletion of IBM1 reduces the steady-state nuclear localization ofHAC1mRNA.HAC1mRNA subcellular localization was analyzed by FISH using Quasar®670-HAC1probes in the indicated strains. The nuclear to cytoplasmic ratio ofHAC1mRNA signal intensity was quantified. As in Fig.4c, Nuclear and cytoplasmic Quasar®670-HAC1signal intensities were measured in at least 200 cells. Unpaired two-tailedt-test (pvalues < 0.0001 forisw1Δ,hac1ΔIBM1 andisw1Δhac1ΔIBM1 strains relative to WT and forhac1ΔIBM1 relative toisw1Δ and toisw1Δhac1ΔIBM1.pvalue 0.6402 forisw1Δhac1ΔIBM 1relative toisw1Δ). Nuclear to cytoplasmic ratio were plotted into whiskers plots. Boxes extend from the 25th to 75th percentiles. The line in the middle of the box is plotted at the median. Whiskers are plotted down to the minimum and up to the maximum value, and each individual value is plotted as a point superimposed on the graph. Two independent experiments were performed with similar results. 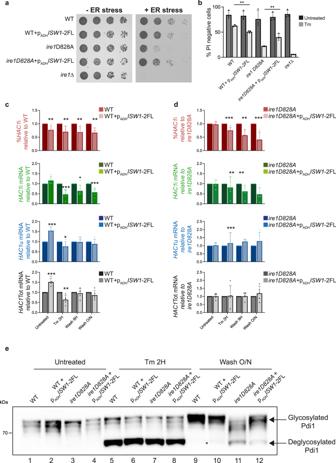Fig. 6: Isw1 overexpression negatively regulates the UPR. aIsw1 overexpression sensitizes WT cells to Tm but partially rescues the growth ofire1D828Acells on Tm. Fivefold serial dilutions of the indicated strains grown for 3 days at 30 °C on selective media containing (+ER stress) or not (−ER stress) 0,4 μg/mL Tm.bViability of the indicated strains was analyzed as described in Fig.3b.n= 3 independent experiments, mean ± sd. Unpaired one-tailedt-tests (pvalues under Tm conditions: WT + pADHISW1−2FL relative to WT: 1.28E−03,ire1D828A+ pADHISW1−2FL relative toire1D828A:5.67E−03).c,dIsw1 overexpression impairsHAC1mRNA splicing. qRT-PCR analysis of the expression levels ofHAC1i,HAC1u, andHAC1Tot relative to WT in the indicated strains.n= 5 independent experiments, mean ± s.d. Unpaired one-tailedt-tests (pvalues %HACi for WT + pADHISW1−2FL relative to WT: 3.23E−03, 5.78E−03, 3.62E−03 and 1.34E−03 for Untreated, Tm 2H, Wash 3H and Wash O/N conditions respectively.pvalues %HACi forire1D828A+ pADHISW1−2FL + pADHISW1−2FL relative toire1D828A: 3.25E−0, 8.76E−04, 1.27E−03 and 8.75E−04 for Untreated, Tm 2H, Wash 3H and Wash O/N conditions respectively).pvalues ofHAC1i,HAC1u andHAC1Tot are shown in the source data file. Unnormalized values shown in Supplementary Fig.7b, c.eIsw1 overexpression improves Pdi1 re-glycosylation inire1D828Acells during Tm UPR time course. Total protein extracts from WT andire1D828Acells overexpressing or not Isw1 and collected during Tm UPR time courses were analyzed by western blot with anti-Pdi1 antibodies. *indicates the persistence of deglycosylated Pdi1. Three independent experiments were performed with similar results. 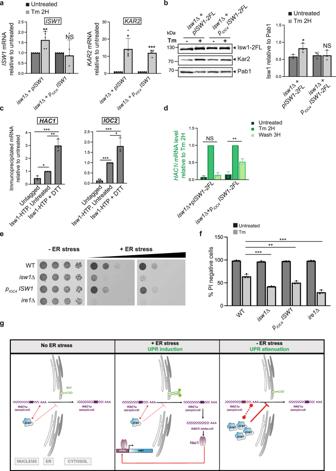Fig. 7: UPR-mediatedISW1induction allows a negative feedback control of the pathway. aSwapping ofISW1endogenous promoter prevents its ER stress induction. Tm-inducedISW1expression is abolished in cells expressing pIOC4ISW1whileKAR2induction is unaffected, as evaluated by qRT-PCR analysis.n= 3 independent experiments, mean ± s.d. Unpaired one-tailedt-tests (pvalues relative to Untreated forISW1target: 4.22E−03 and 3.83E−01 forisw1Δ+pISW1−2FL andisw1Δ+pIOC4ISW1−2FL respectively.pvalues relative to Untreated forKAR2target: 6.94E−04 and 1.70E−07 forisw1Δ+pISW1−2FL andisw1Δ+pIOC4ISW1−2FL respectively).bSwapping ofISW1endogenous promoter prevents the induction of Isw1 by Tm. Total protein extracts fromisw1Δcells expressingpISW1-2FLorisw1Δ+pIOC4ISW1-2FLgrown in the presence (+) or absence (−) of 1 μg/mL Tm for 2 H were analyzed by western blot with anti-FLAG, anti-Pab1 (loading) and anti-Kar2 (UPR induction) antibodies and the level of Isw1 relative to Pab1 was quantified. n = 3 independent experiments, mean ± s.d. Unpaired one-tailedt-tests (pvalues Tm 2 H relative to Untreated: 2.69E−02 and 4.96E−01 forisw1Δ+pISW1-2FLandisw1Δ+pIOC4ISW1-2FLcells respectively).cThe interaction between Isw1 and its mRNA targets is fostered by ER stress. RIP assays in Isw1-HTP cells treated or not with 2 mM DTT for 1 H. Ratio of co-immunoprecipitated RNA to total RNA relative to untreated quantified by qRT-PCR.n= 3 independent experiments, mean ± s.d. Unpaired one-tailedt-tests (pvalues relative to Untreated forHAC1target: 2.77E−03 and 1.12E−03 for Untagged and Isw1-HTP + DTT respectively. (pvalues relative to Untreated forIOC2target: 3.21E−05 and 1.18E−02 Untagged and Isw1-HTP + DTT respectively.pvalues relative to Untagged forHAC1target: 2.77E−03 and 5.65E−04 for Isw1-HTP, Untreated and Isw1-HTP + DTT respectively.pvalues relative to Untagged forIOC2target: 3.21412E−05 and 9.68E−04 for Isw1-HTP, Untreated and Isw1-HTP + DTT respectively).dCells expressing non-UPR-inducibleISW1(pIOC4ISW1) are defective for UPR termination.HAC1inormalized toSCR1mRNA expression during Tm UPR time courses, relative to Tm 2 H, as evaluated by qRT-PCR inisw1Δcells expressingpISW1orisw1Δ+pIOC4ISW1.n= 3 independent experiments, mean ± s.d. Unpaired one-tailedt-tests (pvalues Wash 3 H relative to Untreated: 1.10E−01and 2.56E−03 forisw1Δ+pISW1-2FLandisw1Δ+pIOC4ISW1-2FLcells respectively. Unnormalized values shown in Supplementary Data Fig.8a.eCells deficient for UPR-mediatedISW1induction are more sensitive to Tm than WT. Fivefold serial dilutions of the indicated strains grown in the presence (+ER stress) or absence (−ER stress) of 0.4 μg/mL Tm.fViability of the indicated strains was analyzed as described in Fig.3b.n= 3 independent experiments, mean ± s.d. Unpaired one-tailedt-tests (pvalues relative to WT under Untreated conditions: 4.46E−01, 5.25E−02 and 3.31E−01 forisw1Δ, pIOC4ISW1andire1Δcells respectively.pvalues relative to WT under Tm conditions: 5.19E−04, 6.18E−03 and 3.11E−04 forisw1Δ, pIOC4ISW1andire1Δcells respectively).gModel: Cross-talk between Isw1-mediated nuclear mRNA quality control and the Unfolded protein response. The nuclear export ofHAC1mRNA is restricted by direct binding of the chromatin remodeler Isw1 to its 3′UTR. This nuclear retention activity of Isw1 is reinforced by its UPR induction and appears critical for accurate UPR termination and cell survival upon ER stress. Reporting summary Further information on research design is available in the Nature Research Reporting Summary linked to this article.